Transdifferentiation of parathyroid cells into cervical thymi promotes atypical T-cell development The thoracic thymus is the primary vertebrate organ for T-cell generation. Accessory cervical thymi have also been identified in humans and mice, and shown in mice to be independent functional organs that support T-cell development. However, their origin and functional significance remain unclear. Here we show that cervical thymi in mice have following two origins: delayed differentiation of endodermal precursors and transdifferentiation of parathyroid-fated cells. Compared with thoracic thymus, parathyroid-origin cervical thymi (pCT) express low levels of the thymic epithelial cell-specific transcription factor FOXN1. Consequently, pCT form a distinct microenvironment that supports an atypical thymocyte development pathway, generating T cells with unconventional phenotypic characteristics. Our data demonstrate a transdifferentiation origin for a subset of cervical thymi, with specific functional consequences for T-cell development. In addition to the main, thoracic thymus, cervical thymi (CT) located in the neck have been reported to be present in about 50% of both humans and mice [1] , [2] , and have recently been shown to be a production site for functional T cells that can contribute to peripheral immunity [3] , [4] . CT in mice have also been reported to have an altered tissue-restricted antigen profile, which could lead to the production of autoreactive T cells [3] . Previous reports indicate that cervical thymus in mice are identifiable perinatally [3] , [4] and are frequently associated with the parathyroid and/or thyroid glands [3] , [4] . Further analysis supported a ‘birthdate’ for CT [1] some time after E12.5 (ref. 5 ), which is later than the initiation of thoracic thymus organogenesis at about E11. However, their cellular origin remains unknown. The thymus and parathyroid glands have a common origin from third pharyngeal pouch-derived primordia that separate into distinct organs during morphogenesis [6] . We and others have previously shown that parathyroid cell clusters are also located outside these two organs [7] , [8] ; our data showed that these ectopic parathyroid clusters arise as a normal consequence of organ separation, in both mice and humans [7] . The location and timing of the appearance of CT and their possible functional differences compared with thoracic thymi make it important to determine their cellular origins and the molecular mechanisms controlling their development. In the current study, we show that CT arise from two distinct precursor cell populations, both of which originate from the separation of the third pharyngeal pouch-derived endodermal primordium into distinct thymus and parathyroid organs. We further show that a subset of CT arise from cells previously differentiating as parathyroid, and that this subset generate T cells that are functionally distinct from those made by the thoracic thymus. Thus, the generation and origins of CT have clear consequences for their function and may provide a unique model for understanding the establishment and maintenance of cell fate. Cervical thymus formation requires parathyroid organogenesis We tested whether cervical thymus occurrence correlated with known mechanisms of thymus and parathyroid organ development using a genetic approach. FOXN1 is a transcription factor required for thymic epithelial cell (TEC) differentiation, the loss of function of which causes the nude ( nu ) phenotype [9] . 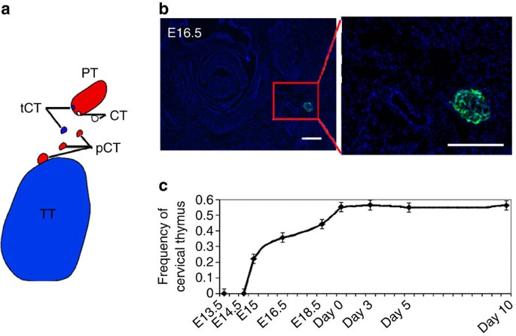Figure 1: The ontology of cervical thymi (CT) and their dependence on parathyroid organogenesis. (a) Schematic of the possible origins of the cervical thymus. Red indicates either parathyroids (PT) or parathyroid-derived CT (pCT); blue indicates thoracic thymus (TT) and thoracic thymus-derived CT (tCT); white indicates non-thymus and non-parathyroid origin for CT. (b) Cervical thymus detected on transverse section of E16.5 Foxn1::EGPF transgenic embryo (green, GFP; blue, 4′,6-diamidino-2-phenylindole (DAPI)). (c) Occurrence of cervical thymus begins at E15 embryonic stage; frequency increases with development until birth (n≥10 for each time point listed) (error bars represent s.e.m.; scale bar, 50 μm). We detected CT by expression of a Foxn1::GFP transgene in newborn Foxn1 nu/nu mice, although they were consistently smaller and present at lower frequency than those in wild-type mice ( χ 2 -test, P =0.0116) ( Table 1 ). We also analyzed Gcm2 null mice, in which all parathyroid cells undergo apoptosis by E12 thus precluding organ separation [7] , for the incidence of CT. No CT were detected among 33 Gcm2 null mutants ( χ 2 -test, P =0.0001) ( Table 1 ). These observations suggest that, like the thoracic thymus, initial cervical thymus formation does not require Foxn1 , while subsequent development and growth does require Foxn1 . However, unlike the thoracic thymus, normal parathyroid organogenesis is required for cervical thymus development. Table 1 Frequency of cervical thymus in neonatal Foxn1 or Gcm2- null mice *. Full size table CT originate in late fetal stages The dependence of cervical thymus development on normal thymus-parathyroid organogenesis suggested three possible origins ( Fig. 1a ). We have shown that the parathyroid domain tends to fragment during normal organ separation and migration, leaving clusters of Gcm2- and parathyroid hormone ( Pth )-positive parathyroid cells between the position of the parathyroid and the thymus after these organs separate [7] . At some frequency, these small clusters of parathyroid cells could be converted to a thymus fate. It is also possible that a few Foxn1 -positive cells are excluded from the encapsulated thymus domain during thymus-parathyroid organ separation. The final possibility is that cells that express neither the Foxn1 nor Gcm2 organ-specific markers within the common thymus-parathyroid primordia are released during organ separation and survive in the neck region, and can be induced by some mechanism to differentiate to a thymus fate. Figure 1: The ontology of cervical thymi (CT) and their dependence on parathyroid organogenesis. ( a ) Schematic of the possible origins of the cervical thymus. Red indicates either parathyroids (PT) or parathyroid-derived CT (pCT); blue indicates thoracic thymus (TT) and thoracic thymus-derived CT (tCT); white indicates non-thymus and non-parathyroid origin for CT. ( b ) Cervical thymus detected on transverse section of E16.5 Foxn1::EGPF transgenic embryo (green, GFP; blue, 4′,6-diamidino-2-phenylindole (DAPI)). ( c ) Occurrence of cervical thymus begins at E15 embryonic stage; frequency increases with development until birth ( n ≥10 for each time point listed) (error bars represent s.e.m. ; scale bar, 50 μm). Full size image Since cervical thymus development occurs later than that of the thoracic thymus [5] , we determined at which stage we could first detect CT, analyzing Foxn1Cre;Rosa26YFP mice from E13.5 until 10 days after birth. The earliest stage at which we detected FOXN1+ cells outside the thoracic thymus was E15, at a frequency of 2/9 embryos, consistent with previously published data that concluded that CT first turn on Foxn1 after E12.5 and before E15.5 (ref. 5 ). The frequency of cervical thymus clusters gradually increased through the later stages of fetal development, reaching a maximum of about 50% at newborn stage ( Fig. 1b,c ). The timing of appearance of Foxn1 -expressing cells in the CT is consistent with their arising from small clusters of Foxn1 -negative cells created by the normal process of thymus-parathyroid separation. A subset of CT originate from parathyroid cells To test whether parathyroid cells might be the origin of CT, we used a parathyroid hormone (Pth)-Cre transgene to activate a fluorescent reporter, tdTomato, and used the Foxn1::EGFP transgene [10] or a FOXN1 antibody to track Foxn1 gene expression. In these mice, parathyroid origin epithelial cells are red (tdTomato+), while Foxn1-expressing thymus cells are green (EGFP+). This Pth-Cre transgene does not have activity in the thoracic thymus ( Supplementary Fig. S1 ). At the newborn stage, two types of CT were observed: those in which cells were doubly positive for both red and green fluorescence ( Fig. 2a,b and Supplementary Fig. S2 ), which we designated as parathyroid-origin CT (pCT) and those with only green fluorescence ( Foxn1 -expressing) ( Fig. 2b,c ). The pCT had a history of parathyroid fate lineage (red) but current Foxn1 expression (green), and had downregulated their parathyroid differentiation program, as indicated by absence of the parathyroid-specific markers Gcm2 and Pth ( Fig. 2d ). 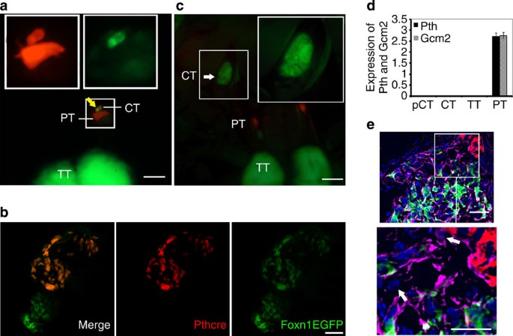Figure 2: Parathyroid origin of a subset of cervical thymi (CT). (a,c) Whole-mount images of 3-day oldPthCre;CAG-td-Tomato;Foxn1::EGPFmice; parathyroid (PT) is red, thoracic thymus (TT) is green. Large boxes show high magnification of CT in small boxes. (Scale bar, 200 μm). (a) CT of parathyroid origin (yellow arrow) next to parathyroid. (b) Section of CT, one with green only, and one with green and red. (Scale bar, 50 μm). (c) Whole-mount image of non-parathyroid origin CT (white arrow). (d) No expression ofPthandGcm2in cervical thymus regardless of origin. (N>3, error bars represent s.e.m.). (e) Epithelial (pankeratin positive) cells at the thymus-parathyroid interface at E12.5 that express neither FOXN1 nor PTH (white arrow).Foxn1::EGPF, green;Pth-Cre-activatedCAG-td Tomato, red; pan-keratin, violet; 4′,6-diamidino-2-phenylindole (DAPI), blue (Scale bar, 50 μm). Figure 2: Parathyroid origin of a subset of cervical thymi (CT). ( a , c ) Whole-mount images of 3-day old PthCre;CAG-td-Tomato;Foxn1::EGPF mice; parathyroid (PT) is red, thoracic thymus (TT) is green. Large boxes show high magnification of CT in small boxes. (Scale bar, 200 μm). ( a ) CT of parathyroid origin (yellow arrow) next to parathyroid. ( b ) Section of CT, one with green only, and one with green and red. (Scale bar, 50 μm). ( c ) Whole-mount image of non-parathyroid origin CT (white arrow). ( d ) No expression of Pth and Gcm2 in cervical thymus regardless of origin. ( N >3, error bars represent s.e.m.). ( e ) Epithelial (pankeratin positive) cells at the thymus-parathyroid interface at E12.5 that express neither FOXN1 nor PTH (white arrow). Foxn1::EGPF , green; Pth-Cre -activated CAG-td Tomato , red; pan-keratin, violet; 4′,6-diamidino-2-phenylindole (DAPI), blue (Scale bar, 50 μm). Full size image Most CT appear to originate from delayed differentiation of endodermal precursors, since about 75% of CT ( Table 2 ) arise from cells that express neither parathyroid markers nor Foxn1 before about E15.5. We will refer to this class as ‘CT’. Consistent with this conclusion, we identified a small number of epithelial cells at the interface between these two organ domains at E12, just before thymus-parathyroid separation that express neither thymus nor parathyroid differentiation markers ( Fig. 2e ). While in the absence of a positive lineage marker we cannot conclusively identify these cells as the source of the non-parathyroid origin CT, their existence is consistent with this model. pCT arise from the transdifferentiation of parathyroid cells, which express Pth at early stages, but subsequently turn off the parathyroid program and switch to a thymus cell fate as shown by Foxn1 expression. We found that CT were broadly distributed between the thyroid and thymus in the neck region, similar to previous reports [3] , [4] . In contrast, most pCT are located near the posterior thyroid, and thus closer to the parathyroid glands proper ( Supplementary Fig. S3 ). Table 2 Frequency of different types of CT at postnatal day 5. Full size table pCT and CT have distinct thymocyte differentiation profiles Given the two different origins for CT, we asked whether their cellular origin influences TEC differentiation and thus the ability to support thymocyte differentiation. We performed flow cytometric analysis of thymocyte differentiation on individual microdissected CT from postnatal day 5 and compared them with newborn and 28-day-old thoracic thymi. About 25% of CT showed an aberrant thymocyte differentiation profile, with a reduced CD4+:CD8+ ratio, and an absence of CD25+ immature thymocytes ( Fig. 3a–d ). This phenotype was confirmed by immunohistochemistry for CD25, which showed variable CD25+ distribution and phenotypes compared with thoracic thymus ( Fig. 4a–i ). Most strikingly, no CD25+ cells could be detected in about 25% of CT ( Fig. 4g–i ). This phenotype was not correlated with organ size, but did track with lineage, as all parathyroid-derived pCT that were assayed for CD25+ thymocytes specifically lacked these cells ( Fig. 4j–m ). In contrast, pCT contain increased frequencies of B, natural killer (NK) and granulocyte populations, while results for CT were similar to thoracic thymus ( Supplementary Fig. S4 ). While CD25+ cells were consistently absent from pCT, the results for CT at postnatal day 5 fell into two categories, either similar to thoracic thymus (see Fig. 3 , CT#1) or very high (CT#2). The frequency of CD25+ cells were consistently anti-correlated with the % of CD4+CD8+ (DP) cells ( Fig. 3c,d ), suggesting that these CT were less well developed. 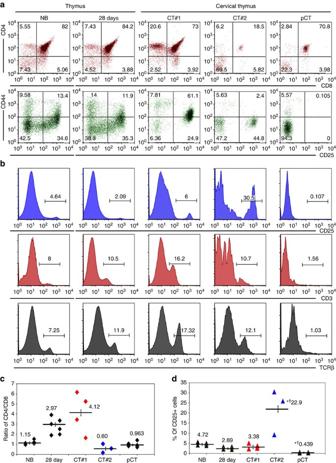Figure 3: Parathyroid-derived cervical thymus support atypical T-cell development. (a) Flow cytometric analysis of thoracic and cervical thymus at postnatal day 3 for CD4, CD8, CD25 and CD44 shows changes in the frequency of thymocyte subsets in CT (N>3). (b) Two classes of CT with either very low CD25 and TCRβ expression, or levels similar to thoracic thymus (N>3). Positive gates are indicated. (c) Ratio of CD4/CD8 is lower in parathyroid-derived cervical thymus but shows variety in non-parathyroid-derived cervical thymus, either similar/higher (CT#1, in red) or lower (CT#2, in blue) compared with thoracic thymus (N>3, error bars represent s.e.m.). (d) Percentage of CD25+ cells is significantly lower in pCT but is significantly higher in the CT#2 group of non-parathyroid-derived cervical thymus (N>3; error bars represent s.e.m., *P<0.01 (significant relative to newborn,t-test);†P<0.01 (significant relative to 28 days,t-test)). Figure 3: Parathyroid-derived cervical thymus support atypical T-cell development. ( a ) Flow cytometric analysis of thoracic and cervical thymus at postnatal day 3 for CD4, CD8, CD25 and CD44 shows changes in the frequency of thymocyte subsets in CT ( N >3). ( b ) Two classes of CT with either very low CD25 and TCRβ expression, or levels similar to thoracic thymus ( N >3). Positive gates are indicated. ( c ) Ratio of CD4/CD8 is lower in parathyroid-derived cervical thymus but shows variety in non-parathyroid-derived cervical thymus, either similar/higher (CT#1, in red) or lower (CT#2, in blue) compared with thoracic thymus ( N >3, error bars represent s.e.m.). ( d ) Percentage of CD25+ cells is significantly lower in pCT but is significantly higher in the CT#2 group of non-parathyroid-derived cervical thymus ( N >3; error bars represent s.e.m., * P <0.01 (significant relative to newborn, t -test); † P <0.01 (significant relative to 28 days, t -test)). 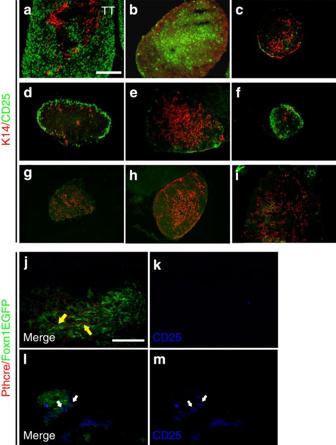Figure 4: Parathyroid-derived cervical thymus cannot support normal T-cell development. (a) CD25+ cells (green) are widespread in E15.5 thoracic thymus and in some cervical thymus (b,c). (d–f) CD25+ cells mainly locate at the sub-capsular area in some CT. (g–i) CD25+ cells are absent in some cervical thymus. (j,k) Parathyroid-derived cervical thymus does not contain CD25+ cells (blue). (l,m) CD25+ cells are present in non-parathyroid-derived cervical thymus (Scale bar, 100 μm). Full size image Figure 4: Parathyroid-derived cervical thymus cannot support normal T-cell development. ( a ) CD25+ cells (green) are widespread in E15.5 thoracic thymus and in some cervical thymus ( b , c ). ( d – f ) CD25+ cells mainly locate at the sub-capsular area in some CT. ( g – i ) CD25+ cells are absent in some cervical thymus. ( j , k ) Parathyroid-derived cervical thymus does not contain CD25+ cells (blue). ( l , m ) CD25+ cells are present in non-parathyroid-derived cervical thymus (Scale bar, 100 μm). Full size image Analysis of T-cell receptor (TCR)β expression further supported these different CT and pCT phenotypes. Thymocytes from pCT consistently had lower frequencies of TCRβ+ thymocytes than those 28-day thoracic thymus, both when measured on total thymocytes and on subsets identified by CD4 and CD8 ( Fig. 3b , Supplementary Fig. S5 and Table 3 ). Reduced TCRβ+ % was seen for all subsets except for CD8 SP, which looked similar to the newborn stage. The levels of TCRβ were also significantly reduced on all subsets except for DPs ( Table 3 ). All CT regardless of CD25+ or DP frequencies have similar TCRβ frequencies on individual subsets, and are generally similar to 28-day controls ( Supplementary Fig. S5 ). However, both CD8+ and CD4−CD8− (DN) subsets displayed higher frequencies of TCRβ+ cells than either newborn or 28-day thymus. The DN expression is particularly interesting and could indicate that either cells have premature TCRβ surface expression or that more mature cells are downregulating their CD4 and/or CD8 expression. As CD3 expression tracked with TCRβ ( Fig. 3b ) and the TCRβ+ DN cells showed a biphasic structure in their levels of TCRβ expression, we lean towards the latter explanation. Table 3 Intensity and frequency of TCRβ expression on cervical thymus-derived thymocytes. Full size table pCT phenotypes are consistent with low Foxn1 expression The thymocyte phenotypes observed in pCT, including selective absence of CD25+ thymocytes, reduced CD4+:CD8+ ratio, reduced TCR levels in the presence of DP and SP thymocytes, and increased frequencies of NK and B cells, are similar to the thoracic thymus phenotypes we previously reported for a severely hypomorphic allele of Foxn1 , Foxn1Δ [11] , [12] , [13] , [14] . Foxn1 hypomorphic alleles result in thymi with a variety of specific and detrimental effects on TEC differentiation and function [11] , [12] , [13] , [14] , [15] , [16] . pCT had fewer FOXN1+ TECs, as well as reduced Foxn1 messenger RNA and protein levels per cell compared with both other CT and thoracic thymus ( Fig. 5a–d ), suggesting that reduced Foxn1 levels suppressed TEC differentiation in pCT and that these defects underlie the thymocytes phenotypes in pCT. Furthermore, CT had average Foxn1 levels that were less than half that of thoracic thymus, although still twice that of pCT ( Fig. 5b,d ). These reduced levels may also underlie the milder but significant differences in thymocyte differentiation in CT. 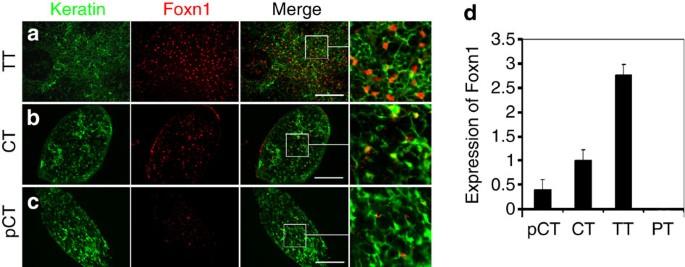Figure 5: Parathyroid-lineage CT have reduced Foxn1 levels at postnatal day 3. (a) FOXN1 in thoracic thymus. (b) FOXN1 in non-parathyroid-derived cervical thymus. (c) FOXN1 in parathyroid-derived cervical thymus is lower than that in non-parathyroid-derived cervical thymus. (d) Real-time PCR analysis ofFoxn1expression in pCT and non-parathyroid-derived (CT) cervical thymus, thoracic thymus (TT) and parathyroids (PT) (N>3, error bars represent s.e.m.) (Scale bar, 50 μm). Figure 5: Parathyroid-lineage CT have reduced Foxn1 levels at postnatal day 3. ( a ) FOXN1 in thoracic thymus. ( b ) FOXN1 in non-parathyroid-derived cervical thymus. ( c ) FOXN1 in parathyroid-derived cervical thymus is lower than that in non-parathyroid-derived cervical thymus. ( d ) Real-time PCR analysis of Foxn1 expression in pCT and non-parathyroid-derived (CT) cervical thymus, thoracic thymus (TT) and parathyroids (PT) ( N >3, error bars represent s.e.m.) (Scale bar, 50 μm). Full size image To determine whether the structure of the thymic microenvironment in CT and pCT was similar to that of Foxn1 hypomorphic thoracic thymi, we analysed the expression of major histocompatibility complex (MHC) class II and binding of the lectin, Ulex europeaus agglutinin 1 (UEA-1), two TEC markers that are significantly reduced in Foxn1 Δ/Δ mice [11] . pCT (parathyroid lineage CT) expressed very low levels of MHC class II and were negative for UEA-1, compared with non-parathyroid-derived CT ( Fig. 6a,b ). This phenotype is similar to that of Foxn1 Δ/Δ mice [11] and is consistent with the thymocyte differentiation defects shown above. These data support the conclusion that parathyroid-derived CT have reduced Foxn1 expression resulting in altered microenvironments, and thus produce thymocytes with functional differences similar to those made by Foxn1 Δ/Δ hypomorphic thoracic thymi, but in wild-type mice. 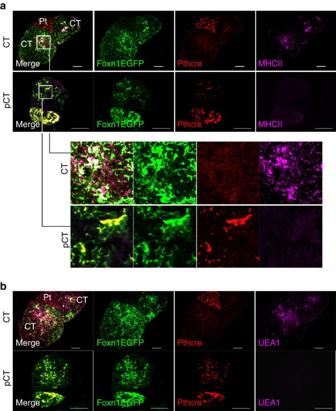Figure 6: Deficient differentiation of epithelial cells in parathyroid-derived cervical thymus. (a) Expression of MHC II in parathyroid-derived cervical thymus (pCT, lower panels) is lower than that in non-parathyroid-derived cervical thymus (CT, upper panels). Higher magnification images of the areas indicated by boxes in the panels inaare shown below panela. (b) UEA-1+ TECs are present in non-parathyroid-derived cervical thymus (CT, upper panel) but not in pCT, lower panel) (Scale bar, 50 μm). Figure 6: Deficient differentiation of epithelial cells in parathyroid-derived cervical thymus. ( a ) Expression of MHC II in parathyroid-derived cervical thymus (pCT, lower panels) is lower than that in non-parathyroid-derived cervical thymus (CT, upper panels). Higher magnification images of the areas indicated by boxes in the panels in a are shown below panel a . ( b ) UEA-1+ TECs are present in non-parathyroid-derived cervical thymus (CT, upper panel) but not in pCT, lower panel) (Scale bar, 50 μm). Full size image Our data present a naturally occurring instance of cell fate switching in vivo , which may be a model for understanding the basis for establishment and maintenance of cell fate. Our results showed that the earliest stage of cervical thymus occurrence is E15–16 days in wild-type mice when CT are very small (<10 cells). After E15, the incidence of cervical thymus gradually increased and reached a maximum of 50% at neonatal and later stages. This gradual increase in incidence suggests that cervical thymus expansion and differentiation is not induced by a single discrete event but may have a stochastic or cumulative element. We did find that absence of Foxn1 can reduce but not eliminate cervical thymus formation and that the CT that do form in nude mice are smaller than that in wild-type mice. Our interpretation of these data is that Foxn1 is required for initial expansion of the cervical thymus, and that in its absence some CT may be too small to detect by these methods or may not persist in the absence of Foxn1 function. Our data clearly show that CT arise as a by-product of normal thymus and parathyroid morphogenesis and show that they can develop via two different differentiation pathways. As CT are absent in mice that lack parathyroids, parathyroid organogenesis is an absolute requirement for cervical thymus formation, even if they derive from delayed differentiation of endodermal precursors. We did identify cells at the thymus-parathyroid junction in the early primordium that express neither thymus nor parathyroid-specific markers. We surmise that these ‘unspecified’ cells are only separated from the thymus during the process of thymus-parathyroid separation—in the absence of the parathyroid, there is no separation, so they would remain encapsulated within the thoracic thymus. As Foxn1 expression is turned on in CT after specification and initial primordium development occurs for the thoracic thymus, we do not have a marker to identify the non-parathyroid-derived cells that form the majority of CT before their expression of Foxn1 , and thus cannot determine whether those cells have acquired a thymus fate or are at this point still unspecified to either organ lineage. Indeed, both types of cells could be present; the two subsets of CT (illustrated by CT#1 and CT#2) could be because of differing origins for these subtypes, namely, whether the cells at the time of activating thymus programme were already specified to a thymus identity, as opposed to being in an unspecified third pouch progenitor condition. In the absence of a molecular marker that identifies thymus-fated cells before Foxn1 expression, we cannot distinguish these possibilities at present. Furthermore, only a subset of parathyroid-fated cells that separate from the main parathyroid convert to the cervical thymus fate. Thus, we cannot at this point easily investigate the initial stages of cervical thymus induction from either cell source. It is possible that differences in the local microenvironments (signaling, matrix components) in which these ectopic clusters are located in addition to differing intrinsic properties of the cell type of origin influence their ability to be induced to a thymus fate. The differing ‘birthdates’ of CT may contribute to the range of phenotypes observed within the non-parathyroid-derived CT. ‘Younger’ CT should look more like fetal stage thymi with few DP cells and many more CD25+ cells (like the CT #2 example), while ‘older’ CT should look more like postnatal thoracic thymi (like the CT #1 example). While it is not possible to know the age of a specific CT on dissection, this explanation does fit with our observation that the frequencies of DP and CD25+ cells are consistently anti-correlated in CT, and with the increasing frequency of CT across late fetal stages, indicating a range of birthdates. Varying Foxn1 levels could also contribute to phenotypic variability; the ability to effectively upregulate Foxn1 could vary with differing mechanisms of activating the program. Our data clearly demonstrate that the phenotype of an individual cervical thymus depends on its cell type of origin; pCT develop by an atypical path, correlated with a lower level of Foxn1. The distinct phenotype of parathyroid-derived pCT (low MHC class II expression, absent UEA-1 staining, selective absence of CD25+ cells, low TCRαβ expression, reversed CD4:CD8 ratio, increased NK and B-cell frequencies) is identical to the phenotype of the Foxn1Δ/Δ hypomorphic allele that we previously reported [11] , [12] , [13] . This T-cell phenotype is also similar to that of ‘T-selected’ CD4 cells in humans, which have been shown to have distinct functional characteristics and may play a discrete protective role relative to other CD4+ T cells [17] , [18] , [19] . Therefore, the pCT can act as a normal source of this specialized subset of T cells that have been proposed to play a unique role in immune function. These results also have potential implications for human immunity, as the presence and type of CT could influence the frequency of this subset of T cells that has been implicated as providing added protection against infectious diseases [20] . Furthermore, patients with Gcm2 mutations [21] should lack both CT and pCT, but specific clinical study of the immune status and phenotypes of these individuals has not been done. The fact that thymi arising from cell fate switching do not completely upregulate their new organ-specific programme also has implications for efforts to develop protocols for cellular reprogramming, including for other endodermal organs such as the liver and pancreas. Mice Male and female mice were analysed at E13.5 to 10 postnatal days. Foxn1:eGFP (enhanced green fluorescent protein) mice were obtained from Dr Thomas Boehm (Max Planck Institute of Immunobiology, Freiburg, Germany). Foxn1Cre [22] and Gcm2-null mutant [23] mouse strains and genotyping protocols have been described previously. Rosa26YFP [24] , Rosa-td-Tomato [25] and PthCre [26] strains were obtained from The Jackson Labs. All mice were genotyped using PCR. 5′-GAGCTGAAGGGCATCGACTT-3′ and 5′-CTTGTGCCCCAGGATGTTG-3′ were used as primers for Foxn1::eGFP, 5′GGACATGTTCAGGGATCGCCAGGCG-3′, 5′-GAGCTGAAGGGCATCGACTT-3′ and 5′-CTTGTGCCCCAGGATGTTG-3′ were used as primers for Foxn1Cre and PthCre , 5′-CACCCTGCCAAATGGTGGATAACA-3′, 5′-CCCTCGCATAAGTCAGCAAACATC-3′, 5′-AAGATGGATTGCACGCAGGTTCT-3′ and 5′-ATCACGGGTAGCCAACGCTATGT-3′ were used as primers for Gcm2 -null, 5′-AAG ACC GCG AAG AGT TTG TC-3′, 5′-AAA GTC GCT CTG AGT TGT TAT-3′ and 5′-GGA GCG GGA GAA ATG GAT ATG-3′ were used as primers for Rosa26YFP, 5′-GAA TTA ATT CCG GTA TAA CTT CG-3′, 5′-AAA GTC GCT CTG AGT TGT TAT-3′ and 5′-CCA GAT GAC TAC CTA TCC TC-3′ were used as primers for Rosa-td-Tomato. All experiments involving animals were approved by the institutional animal care and use committees at the University of Georgia. Messenger RNA analysis from individual thoracic and CT Total RNA from individual cervical and thoracic thymi from 5-day-old C57BL/6 mice was isolated using the RNEasy kit (Qiagen). Complementary DNA was synthesized from the total RNA and used as a template for real-time relative quantitation for Foxn1 (Invitrogen, Mm0043948_m1), Pth (Invitrogen, Mm00451600_g1) and Gcm2 (Invitrogen, Mm00492312_m1) using commercially available reagents (Invitrogen) on an Applied Biosystems 7500 Real Time PCR System. Immunohistochemical procedures Frozen mouse tissues (thoracic and cervical thymus) were sectioned (7 mm) and fixed in 4% formaldehyde in 0.1 M phosphate buffer, pH 7.4 for 5 min at 4 °C or in absolute acetone for 20 s at −20 °C. Tissues were rinsed with PBS, blocked with 10% donkey serum in 0.1 M phosphate buffer, pH 7.4 for 30 min at room temperature, and then incubated with anti-Foxn1 (Santa Cruz, G-20, 1:200), anti-B220 (BD, RA3-6B2, 1:100), anti-cytokeratin (Sigma, C-11, 1:800), anti-CD31 (BD, MEC13.3, 1:100), anti-CD25 (BD, PC61, 1:100), anti-β5t (MBL, PD021, 1:200), anti-CD11c (BD, HL3, 1:100), anti-Aire (Santa Cruz, M-300, 1:200), anti-K5 (Covance, AF138, 1:1,000), anti-K14 (Covance, AF64, 1:1,000) or UEA1 lectin (Vector Labs, X0922, 1:400). In most experiments, the secondary detection was performed with donkey anti-primary species. For Pthcre;td-Tomato;Foxn1::EGFP observation, tissues were fixed in 4% formaldehyde in 0.1 m phosphate buffer, pH 7.4 for 5 min at 4 °C, washed with 5% sucrose/PBS buffer, pH 7.4 for 1 h, 15% sucrose/PBS buffer, pH 7.4 for 1 h and then sectioned. Tissues were examined by fluorescent microscopy. Flow cytometric analysis Thymocytes harvested from individual thoracic and cervical thymus from 5-day-old mice were suspended at 1 × fluorescence activated cell sorting buffer (1 × PBS with 2% BSA and 0.1% NaN3) and incubated with saturating concentrations of the conjugated monoclonal antibodies CD4-Cy5/APC (Biolegend, GK1.5, 1:150), CD8-Cy7/APC (Biolegend, 53-6.7, 1:150), CD25-APC (BD, PC61, 1:150) and CD44-PerCP (Biolegend, IM-7, 1:150), CD3-PE (Biolegend, 145-2C11, 1:150) and TCR- fluorescein isothiocyanate (BD, 0901, 1:150) at 4 C for 30 min, washed, and then fixed with 1% paraformaldehyde (EM Sciences, Ft. Washington, PA) before analysis on a FACS Caliber (Becton Dickinson and Co., San Jose, CA). Statistics Data are presented as the mean and s.e.m. Comparisons between two groups were made using Student’s t test. P <0.05 was considered significant. The χ 2 -test was used to test for associations between nude and wild-type categories or Gcm2 mutants and wild-type. P <0.05 was considered significant. How to cite this article: Li, J. et al. Transdifferentiation of parathyroid cells into cervical thymi promotes atypical T cell development. Nat. Commun. 4:2959 doi: 10.1038/ncomms3959 (2013).